Quantum metrology for gravitational wave astronomy When Galileo Galilei pointed his telescope towards the sky 400 years ago, he discovered events that had never been seen before. In subsequent centuries, a variety of telescopes were invented, covering a large part of the electromagnetic spectrum. These telescopes enabled observations that now form the basis of our understanding of the origin and the evolution of the Universe. Einstein's general theory of relativity, quite often simply 'general relativity' [1] , predicts the existence of a completely different kind of radiation, the so-called gravitational waves (GWs). As electromagnetic radiation is generated by acceleration of charges, so are GWs produced by accelerating mass distributions, such as supernova explosions or binary neutron stars that spiral into each other. GWs may also be emitted by objects that are electromagnetically dark, black holes, for example. Instruments that can directly observe GWs may well be able to 'light up' the dark side of our Universe. The analysis of the waves' spectrum and their time evolution will provide information about the nature of astrophysical and cosmological events that produced the waves. So far, GWs have not been directly observed. Suitable telescopes for GW astronomy are kilometre-scale laser interferometers that measure the distance between quasi-free-falling mirrors. This measurement can be used to infer changes of spacetime curvature. Current GW detectors are already able to measure extremely small changes of distance with strain sensitivity down to the order of 10 −22 . However, quantum physics imposes a fundamental limit on measurement sensitivity, in particular, in terms of photon-counting noise. In the past, the GW signal with respect to the photon-counting noise could only be increased by increasing the light power. Unfortunately, increasing light power will eventually produce measurable quantum radiation pressure noise. In addition it also increases the thermal load inside the detector and is problematic with respect to the concept of overall low noise. Squeezed light avoids these problems by increasing the measurement sensitivity without increasing the light power. The application of squeezed light is a quantum technology. Injected into an interferometer, it entangles the high-power laser fields in the interferometer arms. The photons detected at the interferometer output port are then no longer independent from each other resulting in a reduced, that is, squeezed, photon-counting noise. As the squeezed light technology does not build on an increase in light power, it keeps the thermal load constant and can conveniently be used in conjunction with other future technologies. In particular, it can be combined with cryogenic cooling of interferometer mirrors for reducing mirror surface Brownian motion. Future GW observatories might actually require squeezed laser light in order to make GW astronomy a reality. Recent progress in the generation of squeezed laser light has brought us to the point where quantum metrology will actually find its first application. In this review, we survey the possible astrophysical sources of GWs and the sensitivity issues related to their detection. We briefly examine the detection efforts performed by classical means and show how they have reached their sensitivity limits. We then introduce the concepts of quantum metrology and squeezed light and address how their deployment in next-generation GWs instruments should finally enable direct GW detection. GWs are ripples in spacetime, that is, dynamic changes in space curvature that propagate at the speed of light. According to general relativity, they are transverse and quadrupolar in nature, have two polarization states and are extremely weak. GWs of detectable amplitude cannot be generated on Earth, but a variety of known astrophysical and cosmological sources are predicted to emit gravitational radiation that should reach the Earth with a strength within reach [2] , [3] . Although GWs have not yet been directly observed, their existence is beyond doubt. A binary system of compact objects, such as neutron stars ( Fig. 1 ) or black holes, emits GWs at twice their orbital frequency. The energy carried away by the GWs leads to a precisely predictable decay in the orbital period of the binary. This mechanism was indeed verified to exquisite precision, with observations of the binary pulsar system PSR1913+16 [4] . The discovery is regarded as unequivocal, albeit indirect, proof of the existence of GWs that led to the 1993 Nobel Prize in Physics. 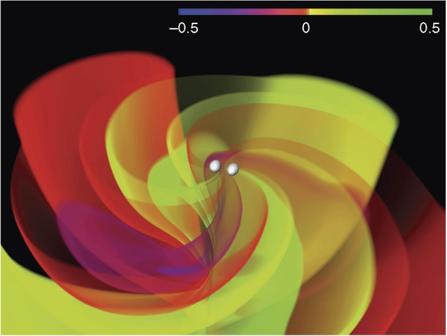Figure 1: Merging neutron stars. Numerical relativity simulation of GWs emitted from two neutron stars6which are about to merge in 4 ms, taken from a movie87. Shown is just the lower half of the sphere. The GW amplitudehis colour coded. At large distances from the stars, the wavelength is given by the distance of two wave fronts having the same colour. The time-resolved detection of these waves including the final merger phase could tell us what is inside neutron stars, that is, their composition and the equation of state of matter at nuclear densities. Reproduced with permission from AEI. Figure 1: Merging neutron stars. Numerical relativity simulation of GWs emitted from two neutron stars [6] which are about to merge in 4 ms, taken from a movie [87] . Shown is just the lower half of the sphere. The GW amplitude h is colour coded. At large distances from the stars, the wavelength is given by the distance of two wave fronts having the same colour. The time-resolved detection of these waves including the final merger phase could tell us what is inside neutron stars, that is, their composition and the equation of state of matter at nuclear densities. Reproduced with permission from AEI. Full size image GWs from complex astrophysical sources carry a plethora of information that will have a major impact on gravitational physics, astrophysics and cosmology. GW signals are typically distinguished in one of the four broad and often overlapping classes [2] , [3] , based on expected waveforms, and hence optimal search techniques. They are binary inspirals and mergers, burst sources, periodic sources, and stochastic sources. In the following, we briefly review the physics and astrophysics that can be extracted from the observation of GWs emitted by these sources. Binary inspirals and mergers The final stages of life of neutron star binaries will provide the richest signals, as shown in Figure 1 . As the binary loses energy, the orbital period decreases and enters the human audio frequency band. After another ≈100 cycles, the stars merge in a catastrophic explosion providing a GW burst signal of a few hundred Hertz up to a kiloHertz. The merger is expected to produce a black hole surrounded by a torus, which will release a giant burst of gamma rays. Simultaneous observation of GWs and gamma rays would confirm that the merger of neutron stars is the engine of many of the observed short, hard gamma ray bursts [5] . Recent advances in numerical relativity now make it possible to make predictions of the waveforms generated around the merger [6] . Comparison with observed waveforms will provide accurate tests of general relativity in the hitherto untested strong-field regime. The imprint of tidal distortions on the GW waveform from a binary system with at least one neutron star will constrain the equation of state of the nuclear matter making up the star. Independent of the nature of the binary, the final state of the merger will be a perturbed black hole, oscillation modes of which will decay in time producing more gravitational radiation. Such observations offer a striking confirmation of the existence of black holes. The famous 'no-hair' theorem says that black holes are completely characterized by their mass and angular momentum [7] . Measuring the GWs emitted by black hole binary systems where the mass ratio of the components is large, the 'no-hair' theorem can be tested. Direct observation of the gravitational waveforms from inspiralling black holes and neutron stars can also provide the luminosity distance to the source without any complex calibrations [2] . If, in addition, the redshift can be measured (via the identification of electromagnetic counterparts), the Hubble parameter [8] , the dark energy and dark matter content of the Universe, and the dark energy equation of state can be determined. Burst sources Burst sources refer to short-lived GW transients, the main known candidates being core-collapse supernovae and collapses to black holes [9] , [10] . Observation of GWs will open a way to extract information about the dynamics occurring in the core of the supernova, and should complement and enhance the understanding gained from electromagnetic observations. Periodic sources Spinning compact objects will generate periodic GW signals depending on the degree of non-axisymmetric deformations [11] (departure from rotational symmetry is a necessary ingredient for generation of quadrupolar moments). Detection of GWs from such sources will confirm models of the underlying physics, which might allow the growth of a 'mountain' on a neutron star. The lack of observation of GWs from the Crab Pulsar at the sensitivity of current ground-based detectors has already constrained its deviation from rotational symmetry [5] . The distribution of neutron stars in the Galaxy could be mapped out using GW observations. Spinning neutron stars currently invisible on Earth could be detected via their GW emission [12] . Stochastic sources Stochastic sources have both astrophysical and cosmological origins [13] , [14] . The 'holy grail' is the Big Bang itself. In principle, we should be able to observe a relic background of GWs from the very early Universe, some time between 10 −18 and 10 −9 s after the Big Bang, when light did not even exist. The electromagnetic analogue of this radiation is the cosmic microwave background, which gives information about conditions in the Universe 385,000 years after the Big Bang [15] , [16] . Gravitational radiation is the only way to observe the conditions in a much earlier epoch. Absence of a detectable stochastic background signal in current GW detectors has constrained certain models of the early Universe on the basis of cosmic superstring population [17] . Of course the most tantalizing sources are those that we do not yet know exist. The opening of every major new electromagnetic window to the Universe has revealed major surprises that have revolutionized our understanding of the Universe. Observing the Universe with an entirely new messenger will very likely continue this tradition. Frequencies of GWs GW astronomy targets phenomena that involve astronomically large masses in acceleration. This, in turn, leads to the expectation that GW emission frequencies will be low, typically below a few tens of kiloHertz. A black hole binary system, for example, has to have an orbital period of just 0.02 s in order to produce GWs at f =100 Hz ( Fig. 2 ). Supernova explosions are expected to have a broad spectral emission, with components that may reach kiloHertz frequencies. However, the strongest detectable GWs are expected at lower frequencies, all the way down to the millihertz or even the nanohertz regime. 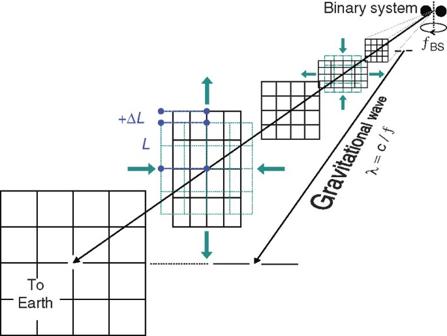Figure 2: GWs are dynamical deformations of spacetime perpendicular to the direction of wave propagation. As a result, distances between free-falling test masses in a transverse plane will change with a strainh=ΔL/L, with quantities defined as shown. For a black hole or neutron star binary system with orbital frequencyfBS, distances will oscillate at twice that frequencyf. The wavelength of this oscillation is given byλ=c/f, withcthe speed of light. Figure 2: GWs are dynamical deformations of spacetime perpendicular to the direction of wave propagation. As a result, distances between free-falling test masses in a transverse plane will change with a strain h =Δ L / L , with quantities defined as shown. For a black hole or neutron star binary system with orbital frequency f BS , distances will oscillate at twice that frequency f . The wavelength of this oscillation is given by λ=c/f , with c the speed of light. Full size image Strength of GWs GWs that reach the Earth are extremely weak. For example, the merger of two neutron stars at the other end of our galaxy ( D ≈50,000 light years away) would produce a GW strain amplitude of about h ≈10 −19 (ref. 2 ). The same source at the distance of about 60 million light years, where the Virgo cluster which comprises up to 2,000 Galaxies are located, would result in a corresponding strain amplitude of only h ≈10 −22 . With the sophisticated technology now available, such tiny strains of spacetime can be detected, and it is very probable that there will be numerous direct detections in the coming decade. Detection using a laser interferometer GWs stretch and compress the spacetime transverse to their direction of propagation. 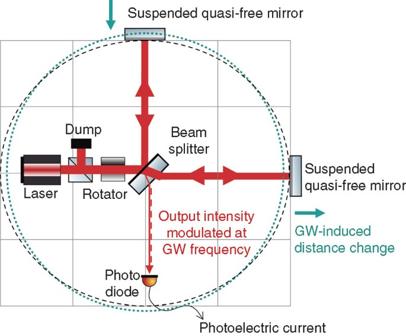Figure 3: Michelson interferometer. Continuous wave laser light is split into two beams travelling in orthogonal directions. Both beams are reflected back towards the central beam splitter. GWs change the optical path length difference, and thus the interference at the beam splitter and the light power directed towards the photo diode. A GW at frequencyfreveals itself as a light power modulation at the same frequency. If the wave was incident on a ring of free test masses in space, in each half cycle of the wave, the ring would distort into an ellipse, as shown in Figure 3 . If the test masses were mirrors, one could reflect laser light off them and observe this GW-induced stretching and compressing of spacetime by measuring the light travel time. This is, in fact, the principle that interferometric GW detectors are based on. An over-view of the history of detectors is given in Box 1 . Figure 3: Michelson interferometer. Continuous wave laser light is split into two beams travelling in orthogonal directions. Both beams are reflected back towards the central beam splitter. GWs change the optical path length difference, and thus the interference at the beam splitter and the light power directed towards the photo diode. A GW at frequency f reveals itself as a light power modulation at the same frequency. Full size image The enormous difficulty of GW detection arises because GWs are expected to be extremely weak when they finally reach the earth. The amount by which a distance L would shrink or stretch due to a GW is proportional to the wave's amplitude h , that is, Δ L = hL . Recalling that we expect strain amplitudes of 10 −22 , we are faced with the prospect of measuring changes in separation of 10 −19 m even for a 1-km interferometer. The intrepid GW detector designer thus faces two categorical challenges. First, how to keep the test masses so still that they respond only to a passing GW rather than to local perturbations? This isolation problem is addressed by techniques of vibration isolation and material engineering, and has to be optimized for the targeted frequency spectrum. Second, how to measure relative displacements with sufficient precision? This measurement problem is tackled by adopting advanced techniques in optical interferometry, control theory and quantum metrology. Let us tackle the question of the mechanical design for an earth-based test mass of spacetime first, followed by a discussion of metrology which launches us into the optical design of the instrument. Box 1: Past and present GW detectors The first experimental attempt to directly measure GWs started in the 1960s [88] . The detection principle was based on the GW-induced resonant excitation of vibrational modes of metal cylinders. Cryogenically cooled devices reached strain sensitivities of about h =10 −18 around a kilohertz, over a band width of a few Hz, in the 1990s and have been further improved since then [89] , [90] , [91] , [92] . Today, the most sensitive instruments are laser interferometers with kilometre size arm lengths. In the past decade, a global network of GW detectors has been realised. The Japanese TAMA project built a 300 m interferometer outside Tokyo, Japan [93] ; the British-German GEO project built a 600 m interferometer near Hannover, Germany [94] , [95] , see Figure 5 ; in the United States, the LIGO project built two 4 km and a 2 km interferometer on sites in Washington and Louisiana [96] , [97] and the European Gravitational Observatory maintains the 3-km-long interferometer Virgo near Pisa, Italy [98] . 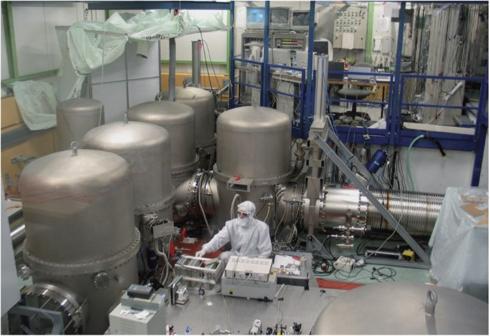Figure 5: GEO 600. View into the central building of the British-German GW detector located close to Hannover, Germany. The vacuum chambers contain the suspended beam splitter, power- and signal-recycling mirrors, additional input and output optics, as well as mirrors to realize a double pass of the laser light through the 600-m-long interferometer arms. Reproduced with permission from the AEI. These detectors target the GW frequency band from 10 Hz to 10 kHz. Currently, the most sensitive detector, LIGO , has achieved a root-mean-square (r.m.s.) strain noise of 3×10 −22 in its most sensitive band from 100 Hz to 200 Hz [96] , thereby reaching its design sensitivity at these frequencies. At such a high sensitivity, detection of GWs is in principle possible. However, an improvement in the sensitivity of GW detectors by about a factor of a hundred is required for GW astronomy. 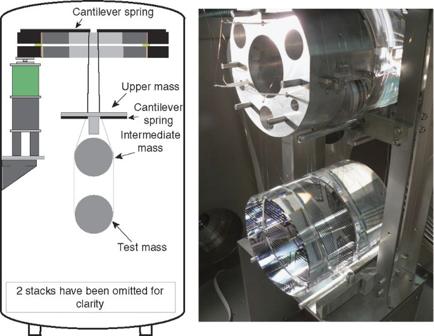Mechanical and optical designs The mirrors of interferometric GW detectors are designed to be quasi-free falling in the directions of propagation of the laser beams, thereby acting as test masses that probe spacetime. Figure 4: Quasi-free-falling test mass. A GW detector requires laser mirrors as test masses in spacetime. Left: Because of the in-vacuum threefold pendulum suspension, the bottom mirror is quasi-free-falling in the direction of laser beam propagation and highly decoupled from the environment. Right: mirrors of today's GW detectors are made of dielectrically coated low absorption-fused silica. Actuated electrostatic forces between the mirror and a reaction mass placed 3 mm behind allow for a stabilization of the interferometer close to its dark fringe. Reproduced with permission from the AEI and the GEO 600 collaboration. This is achieved by suspending the mirrors as sophisticated pendulums in vacuum chambers, as shown in Figure 4 . Above the pendulum's resonant frequency, typically around 1 Hz, the suspension isolates the mirror from vibrations of the ground and the structures on which it is mounted, making it 'quasi-free'. The targeted detection band of earth-based detectors is therefore restricted to the audio band (to frequencies above ≈10 Hz, up to about 10kHz). At lower frequencies, disturbances from the environment are too high, at higher frequencies no strong GW signals are expected, see previous section. Figure 4: Quasi-free-falling test mass. A GW detector requires laser mirrors as test masses in spacetime. Left: Because of the in-vacuum threefold pendulum suspension, the bottom mirror is quasi-free-falling in the direction of laser beam propagation and highly decoupled from the environment. Right: mirrors of today's GW detectors are made of dielectrically coated low absorption-fused silica. Actuated electrostatic forces between the mirror and a reaction mass placed 3 mm behind allow for a stabilization of the interferometer close to its dark fringe. Reproduced with permission from the AEI and the GEO 600 collaboration. Full size image The mirrors and their suspensions are built from materials having exquisitely high mechanical quality factors. This helps to concentrate the thermal energy that causes displacements of the mirror surface into well-defined vibrational frequency modes. At these particular frequencies, no GWs can be detected. The vibrational modes are therefore designed to be outside the detection band for the most part. Ultimately, cryogenic cooling of m may have to be used to further reduce the thermally excited mirror displacement noise, such as those originated from Brownian motion. The first cryogenic interferometric GW detector prototype facilities have been recently realized [18] . A Michelson interferometer—similar to the one used in the Michelson–Morley experiment, which famously established that the speed of light was directionally invariant [19] —is ideally suited to measure the relative light travel time in two orthogonal directions ( Figs 3 and 5 ). In a Michelson interferometer, laser light is incident on a beam splitter that reflects half the light and transmits the other half. Each light beam travels some distance before it is reflected by a mirror back towards the beam splitter where the two beams interfere. The interference provides an output beam, the power of which carries information about the path difference, and GW signals are detected as variations in the light power. Figure 5: GEO 600. View into the central building of the British-German GW detector located close to Hannover, Germany. The vacuum chambers contain the suspended beam splitter, power- and signal-recycling mirrors, additional input and output optics, as well as mirrors to realize a double pass of the laser light through the 600-m-long interferometer arms. Reproduced with permission from the AEI. Full size image It is at this point that quantum physics enters the concept of GW detection. First of all, the light's energy can only be absorbed in discrete quanta (photons), resulting in photon-counting noise or shot-noise. The GW signal-to-shot-noise ratio can in fact be improved by detecting more photons. Shot-noise is proportional to the square root of the number of photons detected, while the mirror displacement signal is directly proportional to the laser power. Consequently, GW detectors use high-power laser systems and optical resonators to maximize their shot-noise-limited sensitivity (for further details, refer to Box 2 ). Fundamentally, there is a second way how the quantum noise of light disturbs a GW detector. The shot-noise inside the interferometer produces a fluctuating radiation pressure force on the test-mass mirrors. The mirrors are randomly displaced by the light, an effect that cannot be distinguished from a GW signal. This is called quantum radiation pressure noise [20] . To reduce this effect, modern GW detectors use test masses of up to 10 kg. As a consequence, radiation pressure noise has not been experimentally observed to date. This situation, however, may change with increasing laser power and is envisioned in the next generation of GW detectors. The design of second-generation GW detectors is more or less completed. These so-called advanced detectors will replace the existing interferometers, aiming for a 10 times increased sensitivity [21] , [22] , [23] . New laser systems will provide up to 200 W of single-mode optical power [24] to reduce quantum shot-noise, yielding a light power of almost a megawatt in the interferometer arm resonators. Larger, 40 kg test-mass mirrors will replace the existing ones to keep the radiation pressure noise low and to allow for larger beam radii to reduce the noise effect of mirror Brownian motion. Cryogenic cooling of test-mass mirrors is another advanced technology that is planned to be implemented in a Japanese detector [18] , [25] . At very cold temperatures, Brownian motion and other forms of thermally excited mirror surface motions (thermal noise) can be significantly reduced. Theoretical modelling of GW sources and estimations of GW event rates [2] suggest that real GW astronomy, with detections on a daily basis with high signal-to-noise ratios, require another 10-fold increased sensitivity for ground-based observatories at frequencies down to a few Hertz. At even lower frequencies, noise on earth is too high and space-based observatories, such as LISA [26] , are required, targeting a frequency spectrum from 10 −4 Hz to about 1 Hz. Above 1 Hz, the Einstein Telescope [27] , [28] is an on-going European design study project for a third-generation ground-based GW detector. An important issue will be the further reduction of the shot-noise (quantum measurement noise), radiation pressure noise acting on the mirrors (quantum back-action noise) and thermal noise. The required reduction of these noise sources poses serious technical challenges. For example, increasing the light power in the interferometer arms will lead to additional absorption and heating of the mirrors. Higher light power will also increase radiation pressure noise. The only classical approach to mitigate noise is, therefore, to use even more massive mirrors. An increased mirror thickness will again lead to increased absorption and heating, making cryogenic cooling of the mirrors impractical. A quantum metrological approach is able to break this vicious circle. In the next section, we will see that squeezed laser light is able to achieve a quantum noise reduction without increasing the light power in a GW detector. Box 2: Signal to shot-noise improvement by classical means In the past decades, several advanced interferometer techniques based on optical resonators were invented to further increase the signal-to-shot-noise ratio in GW detectors. Generally, GW detectors are operated close to a dark fringe, that is, the steady state mirror separation is arranged for nearly perfect destructive interference on the photo diode. This operation point not only cancels common mode noise such as laser noise, but also maximizes the signal to shot-noise ratio. Furthermore, as most of the laser power is reflected back towards the laser, a partially reflecting mirror placed between the laser system and the beam splitter resonantly enhances the light power inside the interferometer. This technique is known as power recycling [99] . Similarly, a partially reflecting mirror placed between the output port of the beam splitter and the photodiode can be used to resonantly enhance the GW signal; this is known as signal recycling [100] . Finally, two partially reflecting mirrors placed near the beam splitter turn the Michelson interferometer arms into kilometre scale Fabry-Perot cavities to increase the phase sensitivity of the interferometer by causing the light to interfere multiple times with itself. All these techniques are classical techniques that maximize the signal-to-shot-noise ratio. At frequencies above a few hundred Hertz, shot-noise is still the limiting noise source for GW detectors. 'Metrology' is the science of measurement. At first glance, quantum physics imposes a fundamental limit on metrology and thus imposes a corresponding limit on the sensitivity of GW detectors. A fundamental problem in optical interferometry is the stochastic distribution of photons arriving at the photodiodes. These statistical fluctuations obscure the tiny power variations caused by GW signals. Fortunately, quantum physics also provides a solution to this problem via the concept of quantum entanglement. 'Quantum metrology' uses quantum entanglement to improve the measurement precision beyond the limit set by measurement-counting noise. The first such proposal was made by Caves in 1981 [29] , when he suggested the use of squeezed states of light as an (additional) input for laser interferometric GW detectors. The initial proposal of Caves was motivated by the limited laser power available at the time. Indeed, squeezed states allow for improvement in the sensitivity of a quantum noise-limited interferometer without increasing the circulating laser power. Squeezed states [30] , [31] , [32] , [33] belong to the class of so-called nonclassical states of light. Generally, nonclassical states are those that cannot be described by a classical (positive valued) probability distribution using the coherent states as a basis (the P -representation) [34] . Let us first consider the coherent states. If light in a coherent state is absorbed by a photodiode, mutually independent photon 'clicks' (in terms of photoelectrons) are recorded, a process that is described by a Poissonian counting statistics. Because of quantum mechanics, every individual 'click' is not predictable, but rather the result of a truly random process. If the number of photons per time interval is large ( n ≫ 1), its s.d. 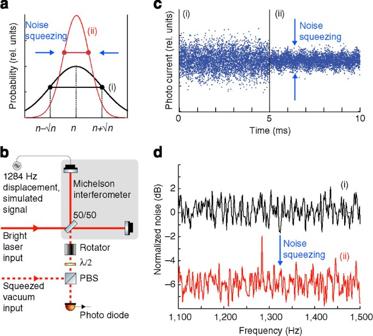Figure 6: Squeezed light-enhanced metrology. (a) For large photon numbersn, squeezed light shows a photon-counting statistic with a s.d. smaller than. In all panels, (i) correspond to shot-noise and (ii) to 6 dB squeezed noise. (b) A squeezed vacuum beam is injected into the dark signal port of a Michelson interferometer, in addition to the conventional bright laser input. The squeezed beam leads to path entanglement of the light fields in the two arms and to an improved signal-to-noise ratio, as shown on the right. Without squeezing, the optical path length modulation at 1284 Hz is visible neither in the time series of the photoelectron current (c, simulation by B. Hage, AEI) nor in its noise power spectrum (d, measurement, image courtesy of H. Vahlbruch, AEI84). In (c) as well as in (d), the signal is clearly visible when squeezing is applied (ii). is given by , as shown in Figure 6a (i). This uncertainty gives rise to shot-noise. For a squeezed light beam, the detection events of photons are not time independent but instead contains quantum correlations. Nevertheless, the photon statistics still cannot be predicted by some external clock. They instead show autocorrelations that give rise to a reduced s.d., as shown in Figure 6a (ii). The correlations might be described in the following way: whenever the quantum statistics might drive the actual photon number above the average value n , a similar number of excess photons destructively interferes with the main body of photons, providing a (partial) compensation for the fluctuation. These quantum correlations squeeze the interferometer's shot-noise below its natural value. Another complementary way of describing the properties of squeezed states is based on the phase space quasi-probability distribution using the amplitude and phase quadratures of a light wave (the Wigner function) [31] , [34] . Figure 6: Squeezed light-enhanced metrology. ( a ) For large photon numbers n , squeezed light shows a photon-counting statistic with a s.d. smaller than . In all panels, (i) correspond to shot-noise and (ii) to 6 dB squeezed noise. ( b ) A squeezed vacuum beam is injected into the dark signal port of a Michelson interferometer, in addition to the conventional bright laser input. The squeezed beam leads to path entanglement of the light fields in the two arms and to an improved signal-to-noise ratio, as shown on the right. Without squeezing, the optical path length modulation at 1284 Hz is visible neither in the time series of the photoelectron current ( c , simulation by B. Hage, AEI) nor in its noise power spectrum ( d , measurement, image courtesy of H. Vahlbruch, AEI [84] ). In ( c ) as well as in ( d ), the signal is clearly visible when squeezing is applied (ii). Full size image A squeezed state that contains only quantum-correlated photons with no coherent amplitude is called a squeezed vacuum state [34] . If such a state is overlapped with a coherent laser beam on a semi-transparent beam splitter, two beam-splitter outputs are generated, which are quantum correlated. As a consequence, the overall (bipartite) quantum state cannot be written in terms of products of the two beam-splitter output states. Such a quantum state is called non-separable or entangled. This is exactly what happens if a squeezed state is injected into the signal output port of a laser interferometer for GW detection ( Fig. 6b ). The two high-power light fields in the interferometer arms get entangled and the light's quantum fluctuations in the two arms are correlated with each other. Although the fluctuations are not predictable from the outside, they provide an improved signal-to-noise ratio in the interferometer. Recall that an interferometer measures the optical path length change in one interferometer arm with respect to the other arm. If the quantum noise in the two arms is correlated, it will cancel out. This entanglement interpretation was not discussed in the initial proposal by Caves. Nevertheless, it shows that the application of squeezed states in interferometers is a real application of quantum metrology by its very own definition. The entanglement produced by splitting a squeezed state at a semi-transparent beam splitter was tomographically characterized and quantified in ref. [35] 35. Figure 6c shows a simulated signal from a photodiode, without (i) and with (ii) squeezing. The tiny modulation in the interferometer's output light due to the (simulated) passing GW is visible only with the improved signal-to-noise ratio. Figure 6d shows the analogue in frequency space, that is, after a Fourier transform of the photocurrent was applied. The above paragraph shows that squeezed states can be conveniently combined with the extremely high photon numbers of coherent light to improve a laser interferometer, as proposed in ref. 29 and shown in Figure 6b . In fact, the stronger the squeezing factor [31] , [34] , the greater the path entanglement and the signal-to-noise improvement. Very strong path entanglement is present in interferometers using so-called NOON-states instead of squeezed states. NOON states are another class of nonclassical states [34] , [36] , [37] , [38] . Unfortunately, the strong entanglement of a NOON state is extremely fragile, in particular if n is large. Very recently, a NOON-state with n =5 photons was demonstrated [38] . However, GW detectors use coherent high-power laser light with n ≈10 23 photons per second. An improvement by the use of NOON states is, therefore, far out of reach. The standard quantum limit (SQL) Shortly after Caves proposed squeezed states of light for laser interferometers in 1981, the first experimental demonstration of squeezed light [39] and proof of principle demonstrations of quantum metrology were achieved [40] , [41] . In parallel, it was theoretically discovered that squeezed states offer even more advances in metrology than 'just' reducing the quantum shot-noise. From the early days of quantum physics, when fundamental aspects of the measurement process were discussed, it was clear that, in general, a measurement disturbs the system that is to be measured [42] . The measurement of quantity A (say a position of a mirror) increases the uncertainty of the non-commuting quantity B (say the mirror's momentum). Both observables are linked by a Heisenberg Uncertainty relation. For repeated measurements of A , the increased uncertainty in B disturbs the measurement of A at later times. This is referred to as quantum back-action noise. Here, the back-action arises from the fluctuating radiation pressure due to the reflected light [20] . It is significant if the mirror's mass is low and a large photon number is reflected. In the 1970s, ideas were developed that showed how, in principle, back-action noise for continuous measurements can be avoided. Such schemes were called quantum non-demolition (QND) measurements [43] , [44] . However, for laser interferometric GW detectors using quasi-free-falling mirrors, it remained unclear whether QND schemes exist. In refs [20] , [29] 20, 29 it was concluded that back-action noise of a free-mass position measurement can in principle not be avoided and, together with photon-counting noise, defines a SQL. In refs [45] , [46] 45, 46, it was argued, however, that measurements below the SQL of a free mass are indeed possible. The discussion remained controversial [47] until Jaekel and Reynaud [48] were able to convincingly show that cleverly arranged squeezed states in a GW detector can simultaneously reduce the shot-noise and the radiation pressure noise, by almost arbitrary amounts (as long as most of the photons belong to the light's coherent displacement). For a summary of QND techniques for free-mass position measurements, we refer to ref. [49] 49. So far no experiment has achieved a position measurement with sensitivity even at, let alone beyond, its SQL. Eventually, this will be achieved, possibly first in future GW detectors. Advanced detectors are in fact designed to have a sensitivity at or very close to their SQLs. Once the SQL is reached, a new level of quantum metrology is achieved, because the position-momentum uncertainty of the mirror becomes correlated with the quadrature uncertainty of the reflected optical field. In this way, entanglement between the mechanical and the optical system can be observed [50] . This is all the more remarkable from the perspective of GW detectors, as we are talking about mirrors with masses of 40 kg, planned for the upcoming improvement to LIGO—the Advanced LIGO [22] . Eventually, even two such mirrors might be projected via entanglement swapping [51] into an entangled state [52] . Obviously, quantum metrology opens the possibility for further studies of the peculiarities of quantum physics at a macroscopic scale. Laser interferometers for GW astronomy are facing extreme sensitivity requirements that can only be achieved if all available tools, inclusive of quantum metrology, are combined in an elaborate measurement device. More recently, squeezed light was also suggested as a resource for quantum information processing [53] , [54] , [55] , [56] . Since then, squeezed light has been central to various proof-of-principle demonstrations, such as quantum teleportation [57] , [58] , and the production of optical 'Schrödinger cat' states for quantum computing and fundamental research on quantum physics [59] , [60] . Squeezed light must be generated in a nonlinear interaction. Squeezed light was first produced in 1985 by Slusher et al . [39] using four-wave mixing in Na atoms in an optical cavity. Shortly after, squeezed light was also generated by four-wave mixing in an optical fibre [61] and by parametric down-conversion in an optical cavity containing a second-order non-linear material [62] . In these first experiments, squeezing of a few percent to 2 to 3 dB were routinely observed (for an overview of earlier experiments and squeezed light generation in the continuous-wave as well as pulsed regime, refer to ref. 63 ). GW detectors are operated with high-power, quasi-monochromatic continuous-wave laser light, with an almost Fourier-limited spatial distribution of a Gaussian TEM 00 mode. For a nonclassical sensitivity improvement, squeezed light in exactly the same spatio-temporal mode must be generated and mode matched into the output port of the interferometer [29] , providing interference with the high-power coherent laser beam at the interferometer's central beam splitter. High-power lasers for GW astronomy are based on optically pumped solid-state crystals in resonators [24] , suggestive of a similar configuration for a 'squeezed light resonator'. 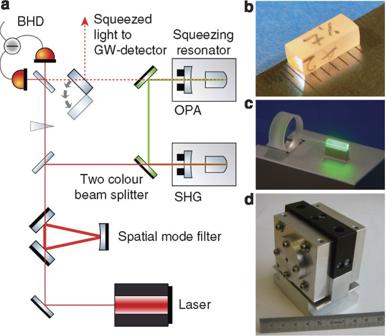Figure 7: Generation of squeezed light. (a) A continuous-wave laser beam at the GW detector wavelength is first spatially filtered and then upconverted to a field at half the wavelength (second harmonic generation, SHG). That beam is then mode matched into the 'squeezing resonator' in which a tiny fraction of the upconverted photons are spontaneously downconverted by optical parametric amplification (OPA) producing a squeezed vacuum state. The squeezing factor is validated by a balanced homodyne detector (BHD). SHG as well as OPA are realized by a nonlinear crystal (b), here a 6-mm-long MgO:LiNbO3crystal, inside an optical resonator (c) formed by an external cavity mirror and the dielectrically coated crystal back surface. The two nonlinear resonators may be constructed in an identical way and are put into temperature stabilized housings (d).b,canddare reproduced with permission from the AEI. Figure 7a shows a schematic setup for generation of squeezed light that is built upon one of the very first squeezing experiments [62] , a setup that has been used in many experiments thereafter [57] , [58] , [64] , [65] . The setup uses a solid-state laser similar to those used as master lasers in high-power systems. After spatial-mode filtering, second harmonic generation in an optical cavity containing a second-order nonlinear crystal is applied to produce laser light at twice the optical frequency. The second harmonic light is then mode matched into the squeezing resonator to pump a degenerate optical parametric amplifier. Figure 7: Generation of squeezed light. ( a ) A continuous-wave laser beam at the GW detector wavelength is first spatially filtered and then upconverted to a field at half the wavelength (second harmonic generation, SHG). That beam is then mode matched into the 'squeezing resonator' in which a tiny fraction of the upconverted photons are spontaneously downconverted by optical parametric amplification (OPA) producing a squeezed vacuum state. The squeezing factor is validated by a balanced homodyne detector (BHD). SHG as well as OPA are realized by a nonlinear crystal ( b ), here a 6-mm-long MgO:LiNbO 3 crystal, inside an optical resonator ( c ) formed by an external cavity mirror and the dielectrically coated crystal back surface. The two nonlinear resonators may be constructed in an identical way and are put into temperature stabilized housings ( d ). b , c and d are reproduced with permission from the AEI. Full size image Figure 7b–d shows photographs of the nonlinear crystal, the optical arrangement and the housing of a squeezing resonator. The crystal is temperature stabilized at its phase-matching temperature. At this temperature, the first-order dielectric polarization of the birefringent crystal material with respect to the pump is optimally overlapped with the second-order dielectric polarization of the resonator mode at the fundamental laser frequency. This ensures a high energy transfer from the pump field to the fundamental Gaussian TEM 00 resonator mode, that is, efficient parametric down-conversion. Initially, the resonator mode is not excited by photons around the fundamental frequency, that is, it is in its ground state, characterized by vacuum fluctuations due to the zero point energy [34] . Note that the process is typically operated below oscillation threshold in order to reduce the phase noise coupling from the pump [66] . This setup produces a squeezed vacuum state [34] . The down-converted photon pairs leaving the squeezing resonator exhibit quantum correlations which give rise to a squeezed photon-counting noise when overlapped with a bright coherent local oscillator beam. The squeezed field is detected by interfering it with a coherent local oscillator beam, either in a balanced homodyne detector, see Figure 7a , or when injected into a GW detector and detected with a local oscillator from the GW detector along with an interferometric phase signal, see Figure 6b . The closer the squeezing resonator is operated to its oscillation threshold, and the lower the optical loss on down-converted photon pairs, the greater the squeeze factor is. For instance, the observation of a squeezing factor of 2 is only possible if the overall optical loss is <50% [63] . A 90% nonclassical noise reduction, that is, a squeezing factor of 10, or 10 dB, already limits the allowed optical loss to <10%. Although squeezed light was demonstrated in the 1980s shortly after the first applications were proposed [39] , [61] , [62] , several important challenges pertaining to the application of squeezed states to GW detectors remained unsolved until recently. First, squeezing had always been demonstrated at Megahertz frequencies, where technical noise sources of the laser light are not present. At these frequencies, the laser operates at or near the shot-noise limit. In the 10 Hz to 10 kHz band where terrestrial GW detectors operate, technical noise masked and overwhelmed the observation of squeezing. For example, the laser relaxation oscillation as well as acoustic disturbances and thermal fluctuations can be many orders of magnitude larger than shot-noise. Until recently, it was not certain that a laser field could even be squeezed and matched to the slow oscillation period of GWs. Second, it was previously not known whether squeezed light was fully compatible with other extremely sophisticated technologies employed in GW detectors, such as signal recycling. Third, the technology to reliably produce stable and strong squeezing with large squeeze factors was lacking. Long-term observation of strong squeezing was a technical challenge until recently. These challenges have all been overcome in the past decade. All the open questions have now been satisfactorily addressed. This development is very timely as many known advanced classical interferometric techniques have almost been exhausted. Many remaining classical improvements are becoming increasingly difficult and expensive to implement. Generation of squeezing in the audio band A major breakthrough in achieving squeezing in the audio band was the insight that the dominant noise at audio frequencies that degrade squeezed light generation couples via the coherent laser field that was used to control the length of the squeezed light laser resonator, whereas noise coupling via the second harmonic pump field is insignificant [67] , [68] . 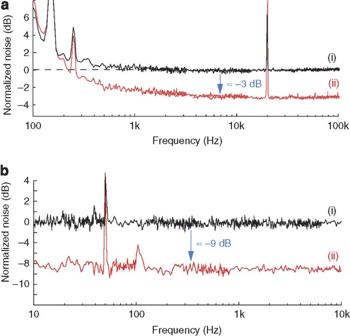Figure 8: Quantum noise squeezing. Both panels show the spectral analysis of measured noise powers without (i) and with ‘squeezing’ (ii). The horizontal sections of traces (i) correspond to shot-noise, serving as reference levels (0 dB), respectively. (a) The first audio-band squeezing down to about 200 Hz was demonstrated by McKenzieet al.in 200469. Reproduced, with permission, from ref.69(©2004 American Physical Society). (b) Current best performance of a squeezed light laser for GW detection shows an up to 9 dB squeezed noise over the complete detection band of ground-based GW detectors85. Reproduced, with permission, from ref.85. This led to the first demonstration of audio band squeezing at frequencies down to 200 Hz [69] , see Figure 8a . There, the length of the squeezing resonator was stabilized without a bright control beam by using the phase sensitivity of the squeezing itself—a technique known as quantum noise locking [70] . Subsequently, a coherent beam control scheme was invented [71] for simultaneous control of both the squeezing resonator length and the squeezing angle [34] . Shortly thereafter another noise source was identified and mitigated, which allowed for squeezing of more than 6 dB throughout the audio band down to 1 Hz [72] . This noise source arose because of tiny numbers of photons that were scattered from the main laser beam and were rescattered into the audio band squeezing mode after having experienced a frequency shift due to vibrations and thermal expansions of potential scattering surfaces, an effect known as parasitic interferences. As bright laser beams cannot be completely avoided, the recipe for the generation of audio band squeezing turned out to be fourfold: avoid scattering by using ultraclean super-polished optics, avoid rescattering by carefully blocking all residual faint beams caused by imperfect anti-reflecting surfaces, reduce the vibrationally and thermally excited motion of all mechanical parts that could potentially act as a re-scattering surface and avoid pointing fluctuations [73] . Figure 8: Quantum noise squeezing. Both panels show the spectral analysis of measured noise powers without (i) and with ‘squeezing’ (ii). The horizontal sections of traces (i) correspond to shot-noise, serving as reference levels (0 dB), respectively. ( a ) The first audio-band squeezing down to about 200 Hz was demonstrated by McKenzie et al. in 2004 [69] . Reproduced, with permission, from ref. [69] (©2004 American Physical Society). ( b ) Current best performance of a squeezed light laser for GW detection shows an up to 9 dB squeezed noise over the complete detection band of ground-based GW detectors [85] . Reproduced, with permission, from ref. [85] . Full size image Compatibility of squeezing with other interferometer techniques Current detectors achieve their exquisite sensitivity to GWs because of their kilometre-scale arm lengths, the enormous light powers circulating in the enhancement resonators (arm, power- and signal-recycling cavities) and sophisticated pendulum suspensions that isolate the test-mass mirrors from the environment ( Figure 3 ). When these techniques were developed, squeezing was not envisioned to become an integrated part of such a system. Building on existing theoretical work [74] , [75] , a series of experimental demonstrations of squeezed state injection into GW detectors were carried out. These included compatibility with power recycling, signal recycling [76] , [77] and with the dynamical system of suspended, quasi-free mirrors [78] , [79] . Generation of strong squeezing Squeezing has significant impact in quantum metrology if large squeezing factors can be produced. Squeezing of 3 dB improves the signal-to-noise ratio by a factor of , equivalent to doubling the power of the coherent laser input. Squeezing of 10 dB corresponds to a 10-fold power increase. Remarkably, the experimentally demonstrated squeezing factors have virtually exploded in recent years [80] , [81] , [82] , culminating in values as large as 12.7 dB [83] . All the squeezing factors above 10 dB were observed with monolithic resonators and at MHz frequencies. However, reduced optical loss in non-monolithic resonators and a careful elimination of parasitic interferences should in principle enable such factors also in the GW band. An 8 to 10 dB improvement based on strong squeezing seems realistic for future GW detectors in their shot-noise-limited band [83] . The first squeezed light laser for GW detection On the basis of the previous achievements reviewed here, very recently, the first squeezed light laser for the continuous operation in GW detectors was designed and completed [84] , [85] . Up to 9 dB of squeezing over the entire GW detection band has been demonstrated ( Figure 8b ). This laser produces squeezed vacuum states and is fully controlled via co-propagating frequency-shifted bright control beams. This 9 dB squeezing factor is limited by technical effects: the squeezing resonator has to have an adjustable air gap to allow for an easy way to apply length control. The anti-reflection coated surface in the resonator introduces additional loss and reduces the escape efficiency. Moreover, a Faraday isolator has to be used in the squeezed beam path in order to eliminate parasitic interferences. This rotator produces a single-pass photon loss of about 2%. This squeezed light source is designated for continuous operation in the GEO600 GW detector. A squeezed light source based on a design that should have less sensitivity to retro-scattered light [86] is being prepared for deployment on one of the most sensitive detectors, the 4 km LIGO detector in Hanford, Washington. The final test of the squeezed light technology for GW astronomy can be carried out only in a (large scale) GW detector. During operation, such a detector takes data 24 h a day, 7 days a week, and future experiments will test appropriate electro-optical auto-alignment systems that continuously provide a high interference contrast between the extremely dim squeezed laser mode and the high-power laser mode at the interferometer's central beam splitter. We are convinced that these experiments will be successful thereby establishing quantum metrology as a key technology for all next generations of GW detectors. As squeezed light builds on quantum correlations between photons, loss of photons reduces the squeezing effect. Future research therefore has to deal with a reduction of photon loss in GW detectors down to a few percent in order to be able to make use of the full potential of squeezed laser light. State of the art optical technologies are already able to provide such low loss. With a sufficiently reduced optical loss also, the enhancement of the nonclassical noise suppression of squeezed light lasers is expedient again thereby preparing the ground for an even higher level of quantum noise reduction. When targeting signal frequencies at which quantum shot-noise is dominating, squeezing will certainly be combined with further increased light powers. When targeting frequencies at which thermal noise and technical noise sources dominate, such as photon scattering, the squeezed light technology will be embedded in a comprehensive low-noise concept providing a new and versatile starting point. This will enable the combination of low shot-noise, QND techniques and the cryogenic operation of mirror test masses, thereby helping to make GW astronomy a reality. How to cite this article: Schnabel, R. et al . Quantum metrology for gravitational wave astronomy. Nat. Commun . 1:121 doi: 10.1038/ncomms1122 (2010).